Venous endothelin guides sympathetic innervation of the developing mouse heart The mechanisms responsible for establishing correct target innervation during organ development are largely unknown. Sympathetic nerves follow blood vessels—typically arteries—to reach their endorgans, suggesting the existence of vascular guidance cues that direct axonal extension. The sinoatrial node and the ventricle of the heart receive sympathetic innervation from the stellate ganglia (STG). Here we show that STG axons follow veins, specifically the superior vena cavae and sinus venosus, to reach these targets. We find that election of these routes is determined by venous endothelium-derived endothelin-1, acting through its specific receptor Ednra expressed within a subpopulation of STG neurons. Furthermore, we demonstrate that Edn1–Ednra signalling is essential for functional regulation of the heart by sympathetic nerves. Our findings present venous Edn1 as a sympathetic guidance cue, and show how axon guidance mechanisms are coordinated with endorgan morphogenesis. With few exceptions, peripheral innervation patterns are established during embryogenesis and are then maintained unchanged for the rest of life. A fundamental goal in neurodevelopmental biology is to elucidate the mechanisms that account for the establishment of these complex patterns. It is generally held that axonal projections follow guidance cues (both attractive and repulsive) along intermediate pathways in order to reach proper targets, and then rely on survival and growth signals at the endorgan for persistence, elaboration and maturation. Only a limited number of guidance cues are currently known, far less than sufficient to explain the complexity of the nervous system. Furthermore, the developmental logic by which expression of guidance cues is integrated with axonal outgrowth and target tissue morphogenesis so as to achieve specific and proper innervation patterning remains unclear. All sympathetic nerves follow blood vessels to reach target organs, a phenomenon called neurovascular congruence, suggesting the expression of guidance signals by the vasculature. The anterior-most superior cervical ganglia (SCG) are located at the bifurcations of the common carotid arteries, and send projections along the internal and external carotid arteries to various targets in the head and neck. In our previous work, we showed that expression of endothelin Edn3 by neural crest-derived smooth muscle of the external carotid arteries guides projections of the endothelin receptor Ednra-positive subset of SCG neurons to this vascular trajectory [1] . The Ednra-negative populations of the SCG are presumably responsive to other still-unknown guidance cues that promote growth along the internal carotid arteries. The heart primarily receives sympathetic innervation from the stellate ganglia (STG), the second-most anterior pair of sympathetic ganglia located at C7/T1 level. Sympathetic nerves synapse on the sinoatrial (SA) node (the pacemaker of the heart) to increase heart rate, and directly on the myocardium to increase contractility, both via release of noradrenalin. Cholinergic parasympathetic nerves from the hindbrain also synapse on the SA node and counteract sympathetic inputs to maintain baseline heart rate. Imbalance in these opposing components of the autonomic nervous system results in deadly consequences: excessive sympathetic action or decreased parasympathetic action is associated with tachycardia (elevated heart rate), whereas decreased sympathetic input is associated with bradycardia (suppressed heart rate) and inefficient cardiac contraction. Virtually nothing is known of the molecular cues that guide the appropriate subset of sympathetic axons from the STG to the heart. In embryos lacking expression of nerve growth factor [2] , or in embryos where nerve growth factor is not induced in myocardium [3] , [4] , sympathetic axons reach but fail to innervate the heart. Semaphorin 3a is expressed in trabecular myocardium (the luminal layer of myocardium) and functions as a repulsive cue, so that sympathetic axons expressing the receptor neuropilin-1 only innervate the subepicardial (outer) myocardium [5] , [6] . However, the roles of these molecules are in mediating growth and patterning of sympathetic axons that have already reached the heart, and do not explain how such axons first reach this target. Interestingly, even the specific vascular routes by which sympathetic axons reach the heart have not been previously defined in the embryo, and are so complex in the adult that their developmental origins cannot be readily inferred. In this study, we have explored cardiac sympathetic axon guidance in the developing mouse, with the specific intention of identifying common themes used by other sympathetic nerves and unique processes that reflect the unique biology of the heart. In every other known case, sympathetic axons only follow arteries to reach target organs, whereas we unexpectedly find that sympathetic axons from the STG follow veins to reach and innervate the SA node and ventricular myocardium. This strategy is coordinated with the developmental derivation of the SA node itself. We demonstrate also that vascular-derived endothelin controls growth and guidance of the STG axons to the heart, a molecular program that in general outline is shared with SCG axons that extend to cranial targets, yet with specific features that reflect the unique developmental and evolutionary logic of the cardiovascular system. Developmental anatomy of cardiac sympathetic innervation To the best of our knowledge, there has been no prior description in any species of how the projection of sympathetic cardiac axons is coordinated with cardiovascular development and maturation. Tyrosine hydroxylase (TH) is a key enzyme in noradrenalin synthesis and is therefore expressed by sympathetic neurons. We used wholemount TH immunostaining of mouse embryonic thoraxes to map the overall structure of the sympathetic ganglia and their projections to the heart. The STG are located bilaterally in the upper thorax, and initiate axonal extension starting around embryonic day E14 ( Fig. 1a,f , Supplementary Fig. 1a ). A large bundle of sympathetic axons from the right STG descends dorsally (with respect to the heart) along the right superior vena cava. At the right sinus horn (the junction of the right vena cava with the sinus venosus; the latter is the common site of venous collection immediately before the right atrium), some of this projection extends laterally to reach the SA node and further extends into the right atrium. The rest of the right STG projection divides into two branches below the sinus horn: one extends laterally to the right and reaches (by E15.5) the right atrium and the lateral wall of the right ventricle, and the other projects laterally to the left and ultimately reaches the lateral wall of the left ventricle ( Fig. 1b,c,g,h,k,l ). The majority of the left STG neurons extend their axons dorsally along the left superior vena cava, the left sinus horn and all the way to the sinus venosus. The sympathetic axons from the left STG that reach the sinus venosus further project onto the dorsal ventricular surface at E15.5 ( Fig. 1c ), and over the next two days continue to grow into large bundles, or are retained as thin fibres, or are pruned ( Fig. 1d ) to establish the final innervation pattern by E17.5 ( Fig. 1e ). 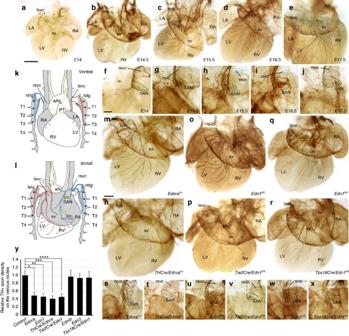Figure 1: Wholemount visualization of STG axonal projections to the heart. (a–e) Developmental progression of mouse cardiac sympathetic axonal growth from the left STGs (dorsal views). Magnified views of the right superior vena cava (grey-dotted line) and the SA node (TH immunoreactive; green-dotted line) ina–eare shown inf–j, visualizing projections from the right STGs. (k,l) Schematic illustration of axonal projections from STG to the ventral surface (k) and the dorsal surface (l) of the heart. Red and blue lines indicate the dorsal projections from the left and right STG, respectively. Orange and turquoise lines denote the ventral projections from the left and right STG, respectively. Yellow lines indicate the projections from SCGs. (m–r) Defective sympathetic innervation of the heart in E15.5 sympathetic neuron-specificEdnra(n) and endothelium-specificEdn1(p) mutants but not in venous smooth muscle/epicardium-specificEdn1mutant (r). (s–x) Magnified views of the right superior vena cava (grey-dotted line) and the SA node (TH immunoreactive; green-dotted line) inm–rshowing reduced projections from the right STG inTHCre/Ednra-(t) andTie2Cre/Edn1(v)-mutant embryos, but not inTbx18Cre/Edn1mutant (x). (y) A compiled representation of sympathetic axon density on the venous routes in E15.5 endothelin signaling component-mutant embryos. For the embryos of each litter, the average fraction of TH-immunostained area in the superior vena cavae and the sinus venosus in control embryos was defined as 1.0. Analysis included results of threeEdnralitters (six controls, sevenEdnra−/−), threeEdnrblitters (six controls, sevenEdnrb−/−), fourEdn1litters (eight controls, sevenEdn1−/−), threeEdn3litters (six controls, eightEdn3−/−), fiveTHCre/Ednralitters (nine controls, nineTHCre/Ednra), fiveTie2Cre/Edn1litters (10 controls, nineTie2Cre/Edn1) and fourTbx18Cre/Edn1litters (eight controls, nineTbx18Cre/Edn1). Error bars; mean ±s.e.m. *P=0.0000001. **P=0.0000000002. ***P=0.00000003. ****P=0.000000001. aAo, ascending aorta; DA, ductus arteriosus; ivc, inferior vena cava; LA, left atrium; lstg, left STG; lsvc; left superior vena cava; LV, left ventricle; PT, pulmonary trunk; RA, right atrium; rstg, right STG; rsvc, right superior vena cava; RV, right ventricle; SAN, SA node; SV, sinus venosus; T, thoracic segment. Scale bars, 500 μm (a–e), 100 μm (f–j,m–r,s–x). Figure 1: Wholemount visualization of STG axonal projections to the heart. ( a – e ) Developmental progression of mouse cardiac sympathetic axonal growth from the left STGs (dorsal views). Magnified views of the right superior vena cava (grey-dotted line) and the SA node (TH immunoreactive; green-dotted line) in a – e are shown in f – j , visualizing projections from the right STGs. ( k , l ) Schematic illustration of axonal projections from STG to the ventral surface ( k ) and the dorsal surface ( l ) of the heart. Red and blue lines indicate the dorsal projections from the left and right STG, respectively. Orange and turquoise lines denote the ventral projections from the left and right STG, respectively. Yellow lines indicate the projections from SCGs. ( m – r ) Defective sympathetic innervation of the heart in E15.5 sympathetic neuron-specific Ednra ( n ) and endothelium-specific Edn1 ( p ) mutants but not in venous smooth muscle/epicardium-specific Edn1 mutant ( r ). ( s – x ) Magnified views of the right superior vena cava (grey-dotted line) and the SA node (TH immunoreactive; green-dotted line) in m – r showing reduced projections from the right STG in THCre/Ednra- ( t ) and Tie2Cre/Edn1 ( v )-mutant embryos, but not in Tbx18Cre/Edn1 mutant ( x ). ( y ) A compiled representation of sympathetic axon density on the venous routes in E15.5 endothelin signaling component-mutant embryos. For the embryos of each litter, the average fraction of TH-immunostained area in the superior vena cavae and the sinus venosus in control embryos was defined as 1.0. Analysis included results of three Ednra litters (six controls, seven Ednra −/− ), three Ednrb litters (six controls, seven Ednrb −/− ), four Edn1 litters (eight controls, seven Edn1 −/− ), three Edn3 litters (six controls, eight Edn3 −/− ), five THCre/Ednra litters (nine controls, nine THCre/Ednra ), five Tie2Cre/Edn1 litters (10 controls, nine Tie2Cre/Edn1 ) and four Tbx18Cre/Edn1 litters (eight controls, nine Tbx18Cre/Edn1 ). Error bars; mean ±s.e.m. * P =0.0000001. ** P =0.0000000002. *** P =0.00000003. **** P =0.000000001. aAo, ascending aorta; DA, ductus arteriosus; ivc, inferior vena cava; LA, left atrium; lstg, left STG; lsvc; left superior vena cava; LV, left ventricle; PT, pulmonary trunk; RA, right atrium; rstg, right STG; rsvc, right superior vena cava; RV, right ventricle; SAN, SA node; SV, sinus venosus; T, thoracic segment. Scale bars, 500 μm ( a – e ), 100 μm ( f – j , m – r , s – x ). Full size image Although most STG cardiac axons project to the dorsal surface of the heart, a very small fraction of the left and right STG projections extend at E15.5 to the ventral (anterior) side of the heart ( Fig. 1k,l ). From the right superior vena cava, these bundles extend to the ascending aorta and descend towards the aortic valve, and then follow the coronary arteries into the myocardium. From the left superior vena cava, sympathetic axons project medially to the ductus arteriosus and the pulmonary trunk, and then cross at valve level to the coronary arteries. The SCG are located at the bifurcation of the internal and external carotid arteries, and project rostrally along these arteries to the head and neck. In addition, a portion of the SCG nerves project caudally along the common carotid arteries towards the heart ( Fig. 1k,l ). By E16.5, these reach the aorta and pulmonary trunk and then intermix on the ventral side of the heart with the ventral projections from the STG. These nerves then become further interconnected and arborized into a wider area and become untraceable from specific ganglia ( Supplementary Fig. 1c ). The SCG nerves do not project to the dorsal side of the heart. These observations reveal several unique features of cardiac sympathetic innervation. First, STG nerves primarily follow venous routes to reach the heart rather than arteries as employed by all other sympathetic nerves elsewhere in the body. Second, there is dramatic asymmetry in target innervation between the left and right STG (for example, the SA node and the lateral ventricular myocardium are exclusively innervated by the right STG, whereas the dorsal ventricular myocardium is primarily innervated by the left STG), which is unique in the sympathetic nervous system. Both observations can be understood in the context of heart morphogenesis (see Discussion). Other than to the heart, STG neurons also extend axons along the subclavian arteries, the intercostal arteries and the vertebral arteries to innervate the forelimbs, the upper thoracic body wall and ribs, and the dorsal side of the neck, respectively. Thus, the STG, like other sympathetic ganglia, contain a heterogeneous population of neurons that extend to several intermediate pathways and reach several final targets. Expression of endothelin components during STG outgrowth We previously showed that vascular smooth muscle-derived endothelins (primarily Edn3), acting through the receptor Ednra, guides the subset of sympathetic axons from the SCG that project along the external carotid arteries [1] . To explore the possibility that endothelin signalling also controls STG axon guidance to the heart, we first examined expression of endothelin signalling components by in situ hybridization during the critical time of STG axonal outgrowth. Both endothelin receptor genes, Ednra and Ednrb , were expressed in distinct subpopulations of STG neurons at E14.5 ( Supplementary Fig. 2a,b ). Triple-stained serial sections of Tie2Cre/R26R lacZ embryos showed that Edn1 and Edn3 were expressed by the endothelium of the left and right superior vena cavae and the sinus venosus, and of their vasa vasora (small capillaries of the large blood vessel wall), in close juxtaposition with TH-immunolabelled STG axons that traverse these vessels (Fig. 2a–f,j–l ). Edn1 and Edn3 were not expressed by the smooth muscle of these vessels. Edn1 and Edn3 were not detected in endothelium or smooth muscle of the ascending aorta ( Supplementary Fig. 2e,i ), which serves as an intermediate route for the small subset of STG and SCG axons that reach the ventral surface of the heart; these pathways may therefore be guided by other factors. Edn2 was undetectable in most of the vascular trajectories for STG neurons ( Fig. 2h–i , Supplementary Fig. 2g ), but was expressed at a low level by endothelial cells of the right superior vena cava ( Fig. 2g ). Edn1 and Edn3 were both expressed by the epicardium and by a subset of cardiomyocytes at E14.5, although sympathetic axons have not reached the heart at this stage. 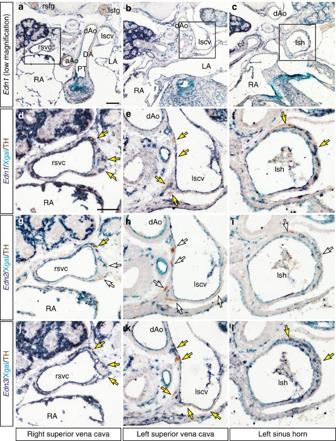Figure 2: Expression of endothelins in the STG vascular routes to the heart. Serial transverse sections of E14.5Tie2Cre/R26RlacZembryo at the level indicated stained with X-gal (blue), immunostained for TH (brown) and labelled byin situhybridization for indicated genes (purple). Yellow arrows point to the juxtaposition of STG axons and endothelin expressing endothelial wall of the venous routes. White arrows denote STG projections along the veins. dAo, descending aorta; lsh, left sinus horn. Scale bars, 100 μm (a–c); 50 μm (d–l). Figure 2: Expression of endothelins in the STG vascular routes to the heart. Serial transverse sections of E14.5 Tie2Cre/R26R lacZ embryo at the level indicated stained with X-gal (blue), immunostained for TH (brown) and labelled by in situ hybridization for indicated genes (purple). Yellow arrows point to the juxtaposition of STG axons and endothelin expressing endothelial wall of the venous routes. White arrows denote STG projections along the veins. dAo, descending aorta; lsh, left sinus horn. Scale bars, 100 μm ( a – c ); 50 μm ( d – l ). Full size image Endothelin signalling controls STG axon guidance to the heart The expression profile of endothelin ligands and receptors is consistent with a role in guiding sympathetic axons to the heart. To directly demonstrate this process, STG axonal projections were assessed by wholemount TH immunostaining in mouse embryos harbouring null mutations in endothelin signalling components. In Ednra- and Edn1 -mutant embryos at E15.5, we observed a substantial disorganization and reduced thickness of STG axonal bundles along the superior vena cavae and the sinus venosus, and in the number of axonal projections to the dorsal side of the heart ( Fig. 1y , Supplementary Fig. 1d–g,l–o ). Sympathetic heart innervation was not completely eliminated, as a minor fraction of sympathetic nerves successfully projected to the dorsal heart surface in these mutants. Projections to the ventral surface of the heart in both mutants were variably compromised, although this is likely to be an indirect consequence of structural cardiac malformations (see below). Although their expression profiles could be consistent with a role in axon guidance, Ednrb- and Edn3 -mutant embryos both exhibited normal STG axonal morphology along the normal venous routes and normal innervation of the dorsal ventricular surface ( Fig. 1y , Supplementary Fig. 1h–k,p–s ). These observations show that Edn1 serves as a guidance cue for Ednra-positive sympathetic axons from the STG to the heart. The analysis of global Ednra and Edn1 mutants is complicated by the presence of unrelated cardiovascular structural phenotypes (VSD, DORV and great vessel defects), craniofacial defects and perinatal lethality in both mutant backgrounds [7] , [8] . These phenotypes result from perturbation of early heart field organization and then later neural crest cell migration and differentiation. We undertook conditional mutagenesis to bypass these issues. We crossed a THCre allele ( Supplementary Fig. 3a,b ) with a conditional Ednra allele to achieve sympathetic neuron-specific receptor mutation, and crossed a Tie2Cre allele with a conditional Edn1 allele to ablate Edn1 production in the vascular endothelial cell lineage. THCre/Ednra and Tie2Cre/Edn1 mutants did not have cardiovascular or craniofacial malformations and survived normally through adulthood. In both conditional mutant backgrounds, we noted a significant decrease in heart innervation ( Fig. 1m–p,s–v , Supplementary Fig. 1b ). Reduced innervation was also evident along the venous trajectories to the SA node and the dorsal ventricular surface, although innervation along the ventral routes was unaffected ( Supplementary Fig. 1t,u ). The severity of disruption of cardiac innervation in these conditional mutants was comparable with that seen in the corresponding global gene mutants. These in vivo results confirm endothelial Edn1 as the signal that guides Ednra-expressing sympathetic axons along the superior vena cavae and the sinus venosus to the heart. THCre/Ednra mutants but not Tie2Cre/Edn1 mutants also had SCG projection phenotypes along the external carotid arteries ( Supplementary Fig. 4b,d ), as predicted based on our previous analysis [1] . Tbx18Cre is active in the epicardium, epicardium-derived coronary smooth muscle and smooth muscle of the sinus venosus and sinus horns ( Supplementary Fig. 3e–h ). There were no abnormalities in general cardiovascular development or in sympathetic innervation of the heart in Tbx18Cre/Edn1 -mutant embryos ( Fig. 1q,r,w–y ). These observations exclude venous and coronary smooth muscle as a source of Edn1 relevant to cardiac sympathetic innervation. Venous Edn1 promotes STG neurite outgrowth in vitro We next undertook STG explant culture to further define the mode of endothelin action in axonal outgrowth. We observed little or no neurite outgrowth from E14.5 wild-type STG explants in the absence of any signal, but robust outgrowth when any of the three endothelins were uniformly added to the collagen matrix of these cultures ( Fig. 3a,e ). This indicates that STG explants, as also shown previously for SCG explants [1] , require instructive signals such as endothelins in order to initiate outgrowth. The response to endothelin required Ednra function, as there was little outgrowth from STG isolated from Ednra -deficient embryos ( Fig. 3b,f ). 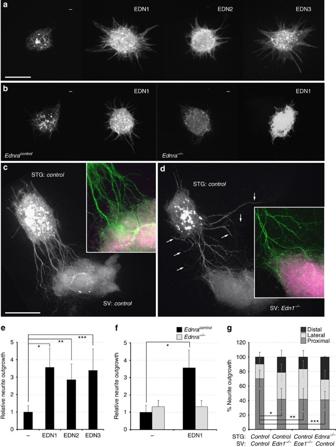Figure 3: Edn1–Ednra signaling is a critical STG axon guidance mechanismin vitro. (a,b) Neurite outgrowths from explanted E14.5 SCGs were visualized by wholemount neurofilament (2H3) staining. (a) Wild-type STG neurite outgrowths in absence or presence of the indicated endothelins (10 nM). A compiled representation of relative neurite outgrowth in the absence (n=16) or presence of EDN1 (n=16), EDN2 (n=16), EDN3 (n=16) is shown ine. (e) Error bars; means±s.e.m.; *P=0.0007, **P=0.002, ***P=0.006. (b) Lack of EDN1 (10 nM) responsiveness inEdnra-deficient STGs. A compiled representation of relative neurite outgrowth fromEdnra−/−(n=10) and littermate control (n=10) STGs is shown inf. (f) Error bars; means±s.e.m.; *P=0.0002. (c,d) Neurite outgrowths from E14.5 STGs cocultured with sinus venosus segment dissected fromEdn1−/−(d) or littermate control (c) embryos were visualized by wholemount TH staining. Arrows denote non-directional (random) outgrowth from STG. High-magnification views of bracketed area show relatively thinner and abnormal morphology of TH+axons (green) and at the vicinity of the 2H8 (CD31)+Edn1-deficient sinus venosus. A complied representation of directional outgrowth from STG in terms of relative neurite outgrowth projecting proximally, laterally or distally to the SV segment is shown ing. For each set of experiment, total neurite outgrowth from STG (sum of all four quadrants) was defined as 100%, and neurite outgrowth in each quadrant is shown as a fraction of total outgrowth. Analysis includes results of control:control (n=10), control:Edn1−/−(n=10), control:Ece1−/−(n=5) andEdnra−/−:control (n=10) pairs. (g) Error bars; means ±s.e.m.; *P=0.0001, **P=0.0005, ***P=0.001. Scale bars, 100 μm (a–d). Figure 3: Edn1–Ednra signaling is a critical STG axon guidance mechanism in vitro . ( a , b ) Neurite outgrowths from explanted E14.5 SCGs were visualized by wholemount neurofilament (2H3) staining. ( a ) Wild-type STG neurite outgrowths in absence or presence of the indicated endothelins (10 nM). A compiled representation of relative neurite outgrowth in the absence ( n =16) or presence of EDN1 ( n =16), EDN2 ( n =16), EDN3 ( n =16) is shown in e . ( e ) Error bars; means±s.e.m. ; * P =0.0007, ** P =0.002, *** P =0.006. ( b ) Lack of EDN1 (10 nM) responsiveness in Ednra -deficient STGs. A compiled representation of relative neurite outgrowth from Ednra −/− ( n =10) and littermate control ( n =10) STGs is shown in f . ( f ) Error bars; means±s.e.m. ; * P =0.0002. ( c , d ) Neurite outgrowths from E14.5 STGs cocultured with sinus venosus segment dissected from Edn1 −/− ( d ) or littermate control ( c ) embryos were visualized by wholemount TH staining. Arrows denote non-directional (random) outgrowth from STG. High-magnification views of bracketed area show relatively thinner and abnormal morphology of TH + axons (green) and at the vicinity of the 2H8 (CD31) + Edn1 -deficient sinus venosus. A complied representation of directional outgrowth from STG in terms of relative neurite outgrowth projecting proximally, laterally or distally to the SV segment is shown in g . For each set of experiment, total neurite outgrowth from STG (sum of all four quadrants) was defined as 100%, and neurite outgrowth in each quadrant is shown as a fraction of total outgrowth. Analysis includes results of control:control ( n =10), control: Edn1 −/− ( n =10), control: Ece1 −/− ( n =5) and Ednra −/− :control ( n =10) pairs. ( g ) Error bars; means ±s.e.m. ; * P =0.0001, ** P =0.0005, *** P =0.001. Scale bars, 100 μm ( a – d ). Full size image We next cocultured STG explants on collagen gels with dissected vascular segments in the absence of exogenous factors. Venous segments isolated from control embryos exhibited strong tropic (attractive) effects and some trophic (random growth) effects on STG neurite outgrowth ( Fig. 3c,g ). Random outgrowth is the consequence of trophic factors (unknown, but not endothelins) that are also expressed by vascular tissues. Edn1 -null venous segments, however, showed a significantly reduced attraction of neurite outgrowth from the STG, and as a result an increase in random outgrowth to distal and lateral directions ( Fig. 3d,g ). We detected an equivalent reduction in directional STG outgrowth towards venous segments when control STGs were cocultured with Ece1 -deficient [9] (no production of any endothelin) vessels and when Ednra -deficient STG were cocultured with control venous segments ( Fig. 3g ). In these experiments, a fraction of neurites grew directionally from the STG to the venous segment even when these tissues were derived from Ednra -mutant or endothelin-deficient embryos, respectively ( Fig. 3g ). This indicates the existence of other attractive cue(s) secreted from the venous tissue that act on other (non-Ednra-expressing) neurons of the STG. This is also a likely explanation for the small subpopulation of STG axons that projected normally to the SA node and ventricle in the absence of Edn1–Ednra signalling ( Fig. 1n,p,y ). Control STG in the explant assay grew directionally towards explanted aortic arch segments; this was unchanged when the STG were from Ednra mutants, or when the arterial tissue was from Ece1 mutants ( Supplementary Fig. 5 ). This indicates that these arterial segments secrete tropic and trophic signals, as do all vascular segments. Because these projections to aortic segments in vitro are endothelin-independent, they likely represent outgrowth by non-Ednra-expressing neurons of the STG. Similarly, in vivo , the minor fraction of STG axons that project to the aorta and then to the ventral heart surface are also not impacted by Ednra or Edn1 mutation and likely also reflect growth by non-Ednra-expressing neurons. Sympathetic dysfunction in endothelin signalling-mutant hearts We found that heart innervation defects observed during the embryonic period persist in postnatal life in both THCre/Ednra and Tie2Cre/Edn1 mutants ( Fig. 4a ), indicating that no other later mechanism compensates the role of endothelin-dependent axon guidance. Despite their reduced sympathetic innervation, these mutants had no obvious defects in growth or behaviour, had normal basal electrophysiological activity ( Fig. 4b ) and had normal cardiac morphology and basal function ( Supplementary Tables 1 and 2 ). In order to address the dependence of proper autonomic heart circuitry on endothelin-dependent sympathetic innervation, we assessed sympathetic action in THCre/Ednra and Tie2Cre/Edn1 mutants by electrocardiography. We challenged 3-week-old mice with amphetamine, which induces noradrenaline release at synaptic terminus [10] , to quantitatively assess endogenous noradrenaline release from sympathetic nerve termini in the heart. THCre/Ednra and Tie2Cre/Edn1 mutants both exhibited a highly blunted inotropic response immediately (within 2 min) after amphetamine injection ( Fig. 4b,c ), indicating that the quantity of noradrenergic axons is greatly diminished in Edn1–Ednra signalling mutants. The small residual response to amphetamine in these mutants is explained by the presence of some STG axons that successfully innervate the dorsal side of the heart ( Fig. 1n,p ). Amphetamine also acts on the adrenal glands to induce adrenaline release, which circulates in the bloodstream to ultimately dominate the local influence of noradrenalin released from sympathetic cardiac nerves. This delayed response (>10 min) was normal in mutant embryos, as expected ( Fig. 4b,d ). Both mutant mouse lines were also normally responsive to the adrenergic receptor agonist isoproterenol ( Fig. 4e ), which acts directly on cardiomyocytes; this demonstrates that the myocardium and conduction system of the heart are unaffected by the diminished sympathetic innervation of these mutants. These results confirm that endothelin signalling is required to establish proper sympathetic innervation of the heart, and thereby for normal autonomic regulation of heart function. 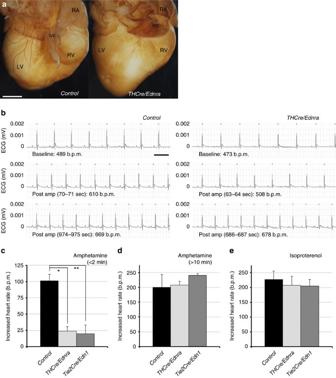Figure 4: Edn1–Ednra signaling mutants exhibit sympathetic dysregulation. (a) Wholemount TH immunostaining visualizing sympathetic innervation of the dorsal surface of hearts from a 3-week-oldTHCre/Ednramutant (right) and a littermate control (left). (b) Representative ECGs from a 3-week-oldTHCre/Ednramutant (right) and a littermate control (left) at the baseline (top) and post-amphetamine administration (middle; <2 min, bottom; >10 min). Green dots denote R-R intervals. (c–e) The change in heart rate following amphetamine (c,d) or isoproterenol (e) administration was measured inTHCre/Ednra(n=5),Tie2Cre/Edn1(n=5) mutants and their controls (n=5) by electrocardiography. Error bars; means ±s.e.m.; *P=0.000001; **P=0.00001. Scale bars, 500 μm (a); 100 ms (b). Figure 4: Edn1–Ednra signaling mutants exhibit sympathetic dysregulation. ( a ) Wholemount TH immunostaining visualizing sympathetic innervation of the dorsal surface of hearts from a 3-week-old THCre/Ednra mutant (right) and a littermate control (left). ( b ) Representative ECGs from a 3-week-old THCre/Ednra mutant (right) and a littermate control (left) at the baseline (top) and post-amphetamine administration (middle; <2 min, bottom; >10 min). Green dots denote R-R intervals. ( c – e ) The change in heart rate following amphetamine ( c , d ) or isoproterenol ( e ) administration was measured in THCre/Ednra ( n =5), Tie2Cre/Edn1 ( n =5) mutants and their controls ( n =5) by electrocardiography. Error bars; means ±s.e.m. ; * P =0.000001; ** P =0.00001. Scale bars, 500 μm ( a ); 100 ms ( b ). Full size image Despite its obvious physiological importance, there has been little understanding of the mechanisms that account for sympathetic innervation of the heart, and how this process is coordinated with heart development. Our results reveal the unexpected utilization of venous routes (the superior vena cavae and the sinus venosus) for guidance of sympathetic axons from the STG to the heart. This developmental strategy is not recognizable from adult heart anatomy because of the complexity of cardiac innervation and because of the incorporation of the sinus venosus into the right atrium in later heart development, and had never before been examined in mouse development. This is the only known example in which sympathetic nerves track along veins rather than arteries to reach their targets, and presumably evolved in response to very specific developmental and/or anatomical constraints. The SA node originates at the junction of the sinus venosus and the atrium on the right dorsal side of the heart. The most direct vascular route to the SA node from outside the heart (i.e., from the STG) is therefore via the right superior vena cava that drains into the sinus venosus. The asymmetrical pattern of STG cardiac projections (right STG primarily to the SA node, left STG primarily to the myocardium) reflects the asymmetry of the developing inflow tract of the heart. In addition to being a more convoluted path, alternate arterial routes to the heart are targets for sensory innervation (chemoreceptive glossopharyngeal nerves sense blood O 2 and CO 2 , and mechanoreceptive vagal nerves sense blood pressure), which may preclude them from serving as sympathetic roadways. Our observations demonstrate that endothelin signalling is the primary axon guidance mechanism that accounts for sympathetic innervation of the SA node and myocardium. Edn1 is expressed by venous endothelium, and serves as a chemoattractive cue for sympathetic axons to project along intermediate targets (the vena cavae and sinus venosus) to reach the heart. It is conceivable that endothelin serves only to initiate axonal growth from the STG toward the vena cavae, and that other venous guidance cues control further extension to the heart, but the observation ( Fig. 2 ) that Edn1 is expressed along the entirety of the venous routes (including the sinus venosus), and the impairment of STG projection to the sinus venosus in vitro when the corresponding tissues lack ligand or receptor ( Fig. 3 ), make this an unlikely model. As described in our previous report, endothelin signalling also guides SCG axons along the external carotid arteries to cranial targets [1] . For the SCG and the STG, the subset of sympathetic ganglia that respond to endothelin cues expresses Ednra. Although Ednrb is expressed by other sympathetic neurons, these do not respond to endothelin ligands and there is no SCG or STG phenotype in Ednrb -mutant mice. Interestingly, the tissue source and type of endothelin differ between the SCG and STG. Guidance of the SCG projections is responsive to Edn3 that is expressed by neural crest-derived vascular smooth muscle; the sharp lineage boundary between the external (neural crest) and internal (mesodermal) carotid artery smooth muscle and the selective expression of Edn3 by the former provides a precise mean of distinguishing these alternate projection pathways. Our initial expectation was that STG innervation to the heart might similarly follow Edn3-expressing neural crest-derived smooth muscle of the ascending aorta and aortic arch; this hypothesis turned out to be incorrect. Arterial guidance of sympathetic neurons by Edn3 is therefore a highly specific property of 3rd arch neural crest for SCG neurons. Our further studies clarify that this specificity is based on temporal grounds. Edn3 is expressed by neural crest-derived smooth muscle of the external carotid arteries, aortic arch and ductus arteriosus (3rd, 4th and 6th arch neural crest, respectively) at E12.5 which then rapidly declines in all vessels by E13.5. The SCG form earliest and initiate projections at E12.5 in response to Edn3 in its vicinity, but the formation of the STG and onset of their axonal projections at E14.0 occur in the absence of Edn3. As we observed in vitro ( Fig. 3a ), STG neurons at E14.5 are competent to respond to Edn3 when it is presented to them. Our studies show that Edn1 is the primary guidance cue for STG innervation of the heart, and our genetic analysis confirms that venous endothelium is the source of this ligand. Edn1 is expressed widely by venous endothelium, and is downregulated in vascular endothelium in response to shear stress such as occurs in arteries [11] , [12] . Thus, Edn1 is a suitable candidate for achieving selective guidance to venous routes. Arterial endothelium is surrounded by a thick layer of vascular smooth muscle in a manner that likely would prevent endothelial cues from reaching nearby ganglia. Thus, in SCG projection to the external carotid arteries, the source of the Edn3 guidance cue is vascular smooth muscle. Arterial routes taken by sympathetic nerves elsewhere in the body presumably also occur in response to various known [13] , [14] , [15] and unknown cues expressed by arterial smooth muscle. In principle, any sympathetic neuron that expresses Ednra should be able to respond to venous Edn1 and extend its axons along veins. Unless other examples exist that have not yet been recognized, this only occurs with STG axons that project to the heart. Several mechanisms might explain this exclusivity. First, sympathetic ganglia exist in a complex environment with multiple tropic and trophic and repulsive factors; venous routes may not be taken in other cases if stronger attractive cues from other vascular targets outcompete the Edn1 signal from venous endothelium. Second, for a neuron to respond to any of these signals, it must express the appropriate receptors, and Ednra-expressing STG neurons might uniquely be nonresponsive to these other signals and thereby only follow a venous route. For lack of a suitable marker that defines Ednra-expressing neuronal axons, we cannot yet determine if the entirety of this population projects to the heart in normal embryos, and if these become rerouted or simply fail to extend in mutant embryos. Tissue-specific mutant mice in our study were anatomically and functionally compromised in heart sympathetic innervation, although were viable and healthy. To explain this observation, we note that the SA node paces heart rate autonomously, and the role of sympathetic innervation is to modulate this activity. Similarly, cardiac contractility is modulated by, but does not require, the release of noradrenaline from sympathetic nerve termini. Even though not required for viability, sympathetic innervation is clearly required for stress response, which we modelled by amphetamine treatment ( Fig. 4 ). The usage of endothelin signalling to establish sympathetic control over heart function would certainly have offered an evolutionary selective survival advantage. In both human and mouse, there are left and right superior vena cavae in early development that drain into the sinus venosus, and the right superior vena cava persists into adulthood in both species. In mice, the left superior vena cava also persists postnatally, and both vena cavae independently empty into the right atrium. In human embryos, the left superior vena cava regresses when the brachiocephalic vein forms de novo as a new conduit between the left jugular vein and the right superior vena cava [16] . This transition occurs after sympathetic innervation patterns to the human heart are already completed [17] . The venous pattern in human and mouse embryos is therefore the same during the critical period when sympathetic innervation is established, which suggests that the same mechanisms are used for establishment of sympathetic circuitry in both species. Animals The THCre [18] , Tie2Cre [19] , Tbx18Cre [20] , R26R [21] , Ednra [8] , Ednrb [22] , Edn1 (ref. 23 ), Edn 3 (ref. 24 ), Ece1 (ref. 9 ), conditional Ednra [25] and conditional Edn1 (ref. 23 ) alleles have been described previously. All experiments with animals complied with National Institute of Health guidelines and were reviewed and approved by the Children’s Hospital Los Angeles Institutional Animal Care and Use Committee. Wholemount TH immunostaining Mouse embryo thoraxes were dissected from paraformaldehyde-fixed embryos, dehydrated by methanol series (50–100%) and incubated overnight in 3% H 2 O 2 in 20% DMSO in methanol solution to quench the endogenous peroxidase activity. Tissues were then rehydrated, and incubated with sheep anti-TH antibody (1:400; Millipore) for 3 days at 4 °C, followed by horse radish peroxidase-conjugated secondary antibody for 3 days at 4 °C. Immunoreactive signal was visualized by DAB detection system. Tissues were dehydrated by methanol series and cleared with benzyl benzoate/benzyl alcohol (2:1). Sympathetic axonal density was quantified by binary threshold-level selection of the TH + area in the superior vena cavae and the sinus venosus area in wholemount digital images using NIS-Element BR software (Nikon). In situ hybridization and immunohistochemistry Glutaraldehyde-fixed embryos were cryopreserved in sucrose. Sixteen-micron cryosections were postfixed, stained with X-gal by standard procedures and then used for in in situ hybridization reactions. Digoxigenin-labelled antisense probes were generated for Edn1, Edn2 and Edn3 (ref. 1 ), and the hybridization signal was detected using an alkaline phosphatase-conjugated anti-digoxigenin antibody and BCIP/NBT (Roche). In situ -labelled sections were then immunolabeled with TH antibody, and visualized using an horse radish peroxidase-conjugated secondary antibody and DAB detection system [1] . Collagen gel explant culture E14.5 STGs were dissected in phosphate-buffered saline, cut into several pieces and placed into a three-dimensional collagen matrix prepared from rat tail collagen (1 mg ml −1 ) [1] . Explants were grown in the absence or presence of 10 nM synthetic endothelins (EDN1, EDN2, EDN3; Enzo Lifescience) in L15CO 2 medium supplemented with 5% fetal bovine serum for 3 days. Neurite outgrowth was evaluated by immunostaining with anti-neurofilament (2H3) (1:100; Developmental Studies Hybridoma Bank) followed by immunofluorescence detection using Alexa Fluor secondary antibodies (Invitrogen). For STG-SV co-culture, E14.5 STGs and sinus venosus segments were separately dissected from Ednra −/− , Edn1 −/− , Ece1 −/− embryos and their littermate controls. Control or Ednra −/− STGs were placed in a collagen gel at the proximity of the sinus venosus segments of the indicated genotype and grown in the same culture medium above for 3 days. Neurite outgrowth was evaluated by immunostaining explants with TH and 2H8 (also known as CD31 or Pecam1) (1:100; Developmental Studies Hybridoma Bank) followed by immunofluorescence detection using Alexa Fluor secondary antibodies (Invitrogen). To quantify neurite outgrowth, the fluorescently labelled neurites extending from explants was measured by binary threshold selection using NIS-Element BR software (Nikon). Electrocardiography Three-week-old mice were anaesthetised by isoflurane inhalation via SomnoSuite small animal anaesthesia system (Kent Scientific), and needle electrodes were inserted subcutaneously with standard lead II arrangement (at the right thoracic limb and the left pelvic limb) to obtain electrocardiography readings with a Powerlab 35 data acquisition system (AD Instruments). Once a stable baseline heart rate was confirmed, drug was administered by intraperitoneal injection. Dosage of drug used was 2 mg kg −1 for amphetamine and 10 ng kg −1 for isoproterenol. The electrocardiography for each subject was recorded continuously for the entire period of the experiment. LabChart 7 software (AD Instruments) was used for heart rate analysis. Ultrasound echocardiography and morphometry Ultrasound echocardiography and morphometry data were obtained by the UCLA physiology core facility. Statistics All quantified data were graphed as mean±s.e.m., and analysed for significance using unpaired Student’s t -test. Minimum sample sizes were determined based on population size, confidence level and s.e. How to cite this article : Manousiouthakis, E. et al. Venous endothelin guides sympathetic innervation of the developing mouse heart. Nat. Commun. 5:3918 doi: 10.1038/ncomms4918 (2014).